Influenza A(H7N9) virus gains neuraminidase inhibitor resistance without loss ofin vivovirulence or transmissibility Without baseline human immunity to the emergent avian influenza A(H7N9) virus, neuraminidase inhibitors are vital for controlling viral replication in severe infections. An amino acid change in the viral neuraminidase associated with drug resistance, NA-R292K (N2 numbering), has been found in some H7N9 clinical isolates. Here we assess the impact of the NA-R292K substitution on antiviral sensitivity and viral replication, pathogenicity and transmissibility of H7N9 viruses. Our data indicate that an H7N9 isolate encoding the NA-R292K substitution is highly resistant to oseltamivir and peramivir and partially resistant to zanamivir. Furthermore, H7N9 reassortants with and without the resistance mutation demonstrate comparable viral replication in primary human respiratory cells, virulence in mice and transmissibility in guinea pigs. Thus, in stark contrast to oseltamivir-resistant seasonal influenza A(H3N2) viruses, H7N9 virus replication and pathogenicity in these models are not substantially altered by the acquisition of high-level oseltamivir resistance due to the NA-R292K mutation. Since the first documented direct transmission of highly pathogenic avian influenza A(H5N1) virus from poultry to humans in the late 1990s, zoonotic influenza A virus infections have been considered to pose a threat to public health. Though all clade 1 and many clade 2 avian H5N1 viruses are resistant to amantadine, the development of neuraminidase (NA) inhibitor resistance in human H5N1 infection has fortunately been rare, and only three oseltamivir-resistant strains have been described [1] , [2] , [3] . On 31 March 2013, Chinese public health authorities reported laboratory confirmation of avian-origin H7N9 influenza virus infections in three people in the greater Shanghai area [4] . Since then, 135 total laboratory-confirmed cases have been reported, resulting in 44 fatalities [5] . Although the source of these infections has not conclusively been confirmed, direct exposure to poultry has been reported in the majority of cases. In consequence, public health authorities closed down poultry markets on 6 April 2013, thus limiting the numbers of new infections [4] . Some live poultry markets began reopening in June under new, stricter infection control standards ( http://www.globaltimes.cn/content/790164.shtml-.Ulw_YII1fo8 ); however, the possibility of avian-to-human transmission still exists. Annual vaccination is still the most effective means of reducing influenza-associated illness and death. However, in the case of a newly emerging influenza virus strain, there is a gap between the epidemic onset and the availability of subtype-specific vaccine supplies, as was seen in the swine-origin H1N1 pandemic in 2009 (ref. 6 ). The prophylactic use of antivirals, particularly in persons at high risk for complicated influenza, can at least partially bridge this gap. Moreover, the timely administration of antivirals to patients severely ill with seasonal, pandemic and avian influenza has been associated with improved clinical outcomes [7] . Two classes of antivirals are available for treatment of acute influenza A virus infection: amantadines and NA inhibitors. For both classes, resistant virus mutants have been described; in fact, treatment of influenza disease currently relies solely on NA inhibitors, because the majority of influenza A and all influenza B isolates infecting humans are resistant to the action of amantadine and rimantadine [7] . The influenza virus NA is a membrane-expressed, glycosylated enzyme with sialidase function, cleaving cell-surface sialic acid receptors to which the haemagglutinin (HA) glycoprotein binds. Its enzymatic activity is critical for the efficient egress of mature viral particles from sialylated host cells, and for the destruction of respiratory tract decoy receptors that impede infection by competing for HA binding [8] . NA inhibitors are sialic acid analogues that block the enzymatic active site and prevent its sialidase activity [9] , and numerous subtype-specific mutations that confer reduced susceptibility to this drug class have been described [10] . Among them, a single nucleotide change in the NA gene can generate resistance to NA inhibitors via an arginine-to-lysine amino acid substitution in the enzymatic active site (R292K in N2 numbering; R294K in N9 numbering [11] ), and this NA-R292K mutation has been reported in patients infected with H7N9 influenza A viruses and treated with NA inhibitors [11] , [12] . However, resistance mutations usually result in a loss in viral fitness, which may be restored by additional compensatory changes in the viral genome [13] , [14] , [15] . Here we investigate whether the R292K-encoding NA of a recent H7N9 clinical isolate confers NA inhibitor resistance and whether it affects the replication or pathogenicity of this strain in primary human tracheobronchial epithelial (hTBE) cell culture and in a mouse virulence model. We also explore the replicative ability of oseltamivir-sensitive and -resistant H7N9 viruses in the lungs of mice treated with oseltamivir or zanamivir, as well as the respiratory droplet transmissibility of these viruses in the guinea pig model. Our results demonstrate that the acquisition of high-level oseltamivir resistance, via the NA-R292K mutation, can significantly impair the sialidase activity of the H7N9 NA without compromising viral replication, virulence or transmissibility in these experimental models. We hypothesize that maintenance of virus fitness is enabled, at least in part, by concurrent, compensatory changes in the expression of HA. The development of oseltamivir resistance, unaccompanied by demonstrable losses of replicative ability in vitro or of virulence or transmissibility in vivo , underscores the multigenic and sometimes unpredictable nature of fitness in influenza A viruses. Susceptibility to NA inhibitors Of the first three influenza A(H7N9) virus isolates collected from Chinese patients (Shanghai/1, Shanghai/2 and Anhui/1), one, Shanghai/1, was found to encode the NA mutation R292K (in N2 numbering, corresponding to residue 294 in the N9 NA). In group 2 NAs, including N2 and N9, this amino-acid substitution has been shown to contribute to decreased susceptibility to NA inhibitors [16] , [17] , [18] , [19] . Thus, we hypothesized that the Shanghai/1-NA would have some degree of inherent resistance to this drug class. To evaluate this prediction experimentally, we generated recombinant A/Puerto Rico/8/1934(H1N1)-based 7:1 reassortant viruses expressing either the Shanghai/1-NA (rPR/8:SH/1-NA) or the Anhui/1-NA (rPR/8:AH/1-NA) by reverse genetics. Using the fluorogenic substrate MUNANA, we calculated the median inhibitory concentration (IC 50 ) at which the NA inhibitors oseltamivir carboxylate, peramivir and zanamivir inhibited 50% of maximal enzymatic activity. 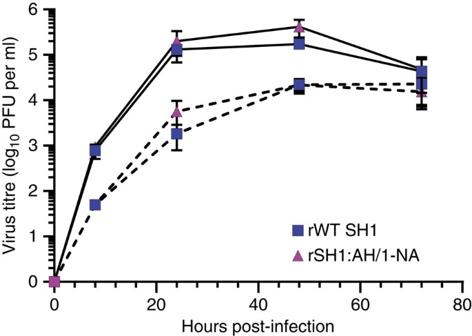Figure 1: Oseltamivir resistance does not affect viral replication in human tracheobronchial epithelial cells. Differentiated human tracheobronchial epithelial cells were infected with rSH/1 (squares) or rSH/1:AH/1-NA (triangles) viruses, at an MOI of 0.01, at either 33 °C (dashed line) or 37 °C (solid line). At 8, 24, 48 and 72 h post infection, cells were washed with PBS/BSA and the concentration of virus in each wash sample was determined by standard plaque assay on MDCK cells. The hTBE growth curves were performed in triplicate. Error bars represent s.d. Compared with the Anhui/1-NA, the Shanghai/1-NA was highly resistant to inhibition by oseltamivir (with a >4,600-fold higher IC 50 ), moderately resistant to peramivir (563-fold higher) and mildly resistant to zanamivir (11-fold higher) ( Table 1 ). Table 1 Resistance of the Shanghai/1-NA to NA inhibitors. 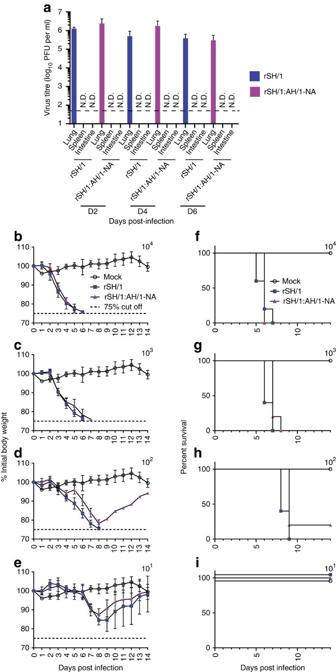Figure 2: Oseltamivir resistance in a recombinantly derived H7N9 virus does not modulate viral pathogenicity in mice. Female BALB/c mice (6–8-week-old) were infected intranasally with various amounts of rSH/1 (squares) or rSH/1:AH/1-NA (triangles) viruses. (a) Viral replication in lung, spleen and intestine. Mice (n=9) were infected intranasally with 100 PFU of rSH/1 (squares) or rSH/1:AH/1-NA (triangles) viruses. On days 2, 4 and 6 post infection, three mice per group were euthanized. The presence of virus in lung, spleen and intestinal tissues was determined by standard plaque assay on MDCK cells. Dashed line indicates the limit of detection (100 PFU ml−1). ND=not detected. (b–e) Weight loss of mice after infection with rSH/1 (squares) or rSH/1:AH/1-NA (triangles) viruses. Mice (n=5) were infected intranasally with serial 10-fold dilutions of each virus, from 104to 101PFU per mouse. The mock animals (circles) were inoculated with PBS/BSA. Following infection, mice were weighed daily, and the average body weights±s.d. of surviving animals in each group up to day 14 post infection are indicated as percentages of the original body weights. Dashed line indicates 75% of initial body weight. (f–i) Survival of mice after infection with rSH/1 (squares) or rSH/1:AH/1-NA (triangles) viruses or mock treated (circles). Kaplan–Meier curves represent survival after infection with each virus at 10-fold dilutions from 104to 101PFU or mock infection with PBS/BSA (n=5 per group). Please note that experimentsb–eandf–ishare the same control mock-infected animals. Error bars represent s.d. in all panels. Full size table NA enzymatic activity and substrate affinity To place these isolates in the context of what is known about the enzymatic activity of oseltamivir-sensitive and -resistant group 2 NAs, we performed MUNANA-based kinetic assays on the 7:1 PR/8 reassortant viruses, normalized to equivalent NA content, to derive the Michaelis–Menten parameters V max and K m ( Table 2 ). Compared with the oseltamivir-sensitive Anhui/1-NA, the oseltamivir-resistant Shanghai/1-NA demonstrated an ~80% reduction in both maximal enzymatic activity ( V max ) and affinity for the MUNANA substrate (1/ K m ). When 7:1 reassortant viruses, diluted to equivalent NA content, were assessed for haemagglutination activity, the haemagglutination unit titre measured for the rPR/8:AH/1-NA virus was two- to fourfold higher than that obtained for rPR/8:SH/1-NA. Thus, relative to oseltamivir-sensitive rPR/8:AH/1-NA, oseltamivir-resistant rPR/8:SH/1-NA displays comparable in vitro reductions in HA receptor binding activity and NA enzymatic function. Table 2 Michaelis–Menten kinetics of the AH/1 and SH/1 NAs. Full size table Virus replication kinetics in hTBE cells To investigate the impact of oseltamivir resistance on the replication of H7N9 viruses, we replaced the oseltamivir-resistant NA of Shanghai/1 with the oseltamivir-sensitive NA of Anhui/1 (rSH/1: AH/1-NA) and compared this virus to recombinant wild-type Shanghai/1 (rSH/1). Efficient replication in the upper respiratory tract is thought to be essential for viral transmission among humans. To assess the effect of oseltamivir resistance on the replication of H7N9 viruses in a relevant primary cell culture model, we infected differentiated hTBE cells with either rSH/1 or rSH/1:AH/1-NA at a multiplicity of infection (MOI) of 0.01, incubated the infected cells at 33 °C or 37 °C, and determined virus titres at 8, 24, 48 and 72 h post infection ( Fig. 1 ). At each temperature, rSH/1 and rSH/1:AH/1-NA showed similar replication kinetics and peak titres, even though both viruses replicated faster at 37 °C than at 33 °C. Thus, our findings indicate that the oseltamivir-resistant NA encoded by A/Shanghai/1 does not compromise the replication of this virus in primary human upper respiratory tract cells. Figure 1: Oseltamivir resistance does not affect viral replication in human tracheobronchial epithelial cells. Differentiated human tracheobronchial epithelial cells were infected with rSH/1 (squares) or rSH/1:AH/1-NA (triangles) viruses, at an MOI of 0.01, at either 33 °C (dashed line) or 37 °C (solid line). At 8, 24, 48 and 72 h post infection, cells were washed with PBS/BSA and the concentration of virus in each wash sample was determined by standard plaque assay on MDCK cells. The hTBE growth curves were performed in triplicate. Error bars represent s.d. Full size image Virus replication in mice Next, we examined the impact of oseltamivir resistance on viral replication in vivo . BALB/c mice were infected with 100 plaque-forming units (PFU) of rSH/1 or rSH/1:AH/1-NA. On day 2, 4 and 6 post infection, virus titres in the lungs of mice were determined ( Fig. 2a ). We observed no significant difference in the replication kinetics of the oseltamivir-resistant isolate (rSH/1) as compared with the oseltamivir-sensitive one (rSH/1:AH/-NA). We also assayed for virus replication in spleen and intestinal tissue; however, no virus was recovered from these extra-pulmonary tissues at any time point ( Fig. 2a ). These findings indicate that the oseltamivir-resistant NA does not compromise virus replication in the lung or alter its tissue tropism in the mouse model. Figure 2: Oseltamivir resistance in a recombinantly derived H7N9 virus does not modulate viral pathogenicity in mice. Female BALB/c mice (6–8-week-old) were infected intranasally with various amounts of rSH/1 (squares) or rSH/1:AH/1-NA (triangles) viruses. ( a ) Viral replication in lung, spleen and intestine. Mice ( n =9) were infected intranasally with 100 PFU of rSH/1 (squares) or rSH/1:AH/1-NA (triangles) viruses. On days 2, 4 and 6 post infection, three mice per group were euthanized. The presence of virus in lung, spleen and intestinal tissues was determined by standard plaque assay on MDCK cells. Dashed line indicates the limit of detection (100 PFU ml −1 ). ND=not detected. ( b – e ) Weight loss of mice after infection with rSH/1 (squares) or rSH/1:AH/1-NA (triangles) viruses. Mice ( n =5) were infected intranasally with serial 10-fold dilutions of each virus, from 10 4 to 10 1 PFU per mouse. The mock animals (circles) were inoculated with PBS/BSA. Following infection, mice were weighed daily, and the average body weights±s.d. of surviving animals in each group up to day 14 post infection are indicated as percentages of the original body weights. Dashed line indicates 75% of initial body weight. ( f – i ) Survival of mice after infection with rSH/1 (squares) or rSH/1:AH/1-NA (triangles) viruses or mock treated (circles). Kaplan–Meier curves represent survival after infection with each virus at 10-fold dilutions from 10 4 to 10 1 PFU or mock infection with PBS/BSA ( n =5 per group). Please note that experiments b – e and f – i share the same control mock-infected animals. Error bars represent s.d. in all panels. Full size image Virulence in mice The attainment of oseltamivir resistance can result in viral attenuation [3] , [19] , [20] . To investigate a potential influence of oseltamivir resistance on virulence of H7N9 viruses in vivo , we determined the median mouse lethal dose (mLD 50 ) of rSH/1 and rSH/1:AH/1-NA. We infected BALB/c mice intranasally with 10-fold serial dilutions of each virus (from 10 4 to 10 1 PFU per mouse), and weight and health status were monitored daily for 14 days post-infection. Mice infected with both viruses demonstrated comparable weight loss patterns ( Fig. 2b–e ) and similar onset of clinical signs of disease, including ruffled fur, hunching and lethargy. The Kaplan–Meier survival curves comparing the two viruses at each inoculating dose were compared by the log-rank test ( Fig. 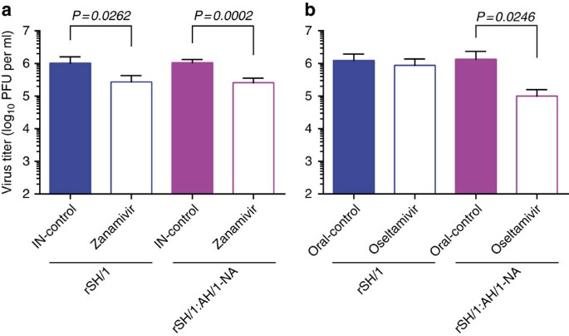Figure 3: Oseltamivir does not suppress H7N9 virus replication in mice infected with rSH/1. Female BALB/c mice (6–8-week-old;n=5) were infected intranasally with 100 PFU of rSH/1 (blue) or rSH/1:AH/1-NA (purple) viruses. Mice were treated with intranasal zanamivir (a), oral oseltamivir (b), intranasal PBS vehicle (a) or oral distilled water vehicle (b) twice daily for 5 days. Five mice were euthanized at day 5 post infection and viral lung titres were determined by plaque assays in MDCK cells. Student’st-test was applied to evaluate the statistical significance between viral titres of control animals and antiviral-treated animals. Error bars indicate s.d. value. 2f–i and Table 3 ). The median time to death in the 10 3 and 10 2 PFU dose groups were slightly longer for rSH/1:AN/1-NA than for rSH/1 ( P =0.0495 and P =0.0442, respectively). However, for the oseltamivir-sensitive virus rSH/1:AH/1-NA we determined an mLD 50 of 42 PFU (95%CI, 10–170 PFU) and for the oseltamivir-resistant virus rSH/1, 32 PFU (95%CI, 8.9–110 PFU), which were not significantly different. Table 3 Median time to death for infected mice. Full size table Viral susceptibility to oseltamivir and zanamivir in mice We further evaluated the in vivo replication of rSH/1 and rSH/1:AH/1-NA in the lungs of mice treated with the NA inhibitors zanamivir and oseltamivir. In the zanamivir treatment group, viral lung titres of both viruses were significantly reduced compared with mice treated with vehicle only ( Fig. 3a ). Virus titres of rSH/1 and rSH/1:AH/1-NA were comparably reduced in zanamivir-treated mice, consistent with the relatively minor 11-fold difference in their in vitro susceptibilities to zanamivir. In contrast, we observed a significant, 1 log reduction in viral lung titres of the oseltamivir-sensitive rSH/1:AH/1-NA virus in mice treated with oral oseltamivir, whereas oseltamivir treatment had no effect on lung titres in mice infected with the oseltamivir-resistant rSH/1 virus ( Fig. 3b ). These results accord with our in vitro observation of the >4,600-fold increase in oseltamivir resistance conferred by the Shanghai/1-NA ( Table 1 ). Figure 3: Oseltamivir does not suppress H7N9 virus replication in mice infected with rSH/1. Female BALB/c mice (6–8-week-old; n =5) were infected intranasally with 100 PFU of rSH/1 (blue) or rSH/1:AH/1-NA (purple) viruses. Mice were treated with intranasal zanamivir ( a ), oral oseltamivir ( b ), intranasal PBS vehicle ( a ) or oral distilled water vehicle ( b ) twice daily for 5 days. Five mice were euthanized at day 5 post infection and viral lung titres were determined by plaque assays in MDCK cells. Student’s t -test was applied to evaluate the statistical significance between viral titres of control animals and antiviral-treated animals. Error bars indicate s.d. value. Full size image Airborne respiratory transmission in guinea pigs Next, we investigated the impact of oseltamivir resistance on airborne respiratory transmission of H7N9 viruses in the guinea pig model. Four guinea pigs were inoculated with rSH/1:AH/1-NA and four with rSH/1. At 1 day post-inoculation, eight naive guinea pigs were exposed to these infected guinea pigs, in cages that precluded direct contact between animals. Transmission events were detected by isolation of infectious influenza virus in the nasal lavage fluid of exposed guinea pigs and confirmed by assessing for H7N9 virus-specific seroconversion ( Table 4 ). The inoculated guinea pigs shed both viruses to similar peak titres with similar timing (10 5 –10 6 PFU ml −1 on day 2 post-inoculation). However, these peak nasal lavage virus titres were, on average, ~1 log lower than those typically observed in guinea pigs inoculated with H3N2 and H1N1 human influenza A isolates [14] , [20] , [21] . Table 4 Airborne respiratory transmission of rSH/1 and rSH/1:AH/1-NA in guinea pigs. Full size table Transmission events were observed in one of four guinea pigs exposed to the oseltamivir-sensitive reassortant rSH/1:AN/1-NA and in two of four guinea pigs exposed to the oseltamivir-resistant recombinant rSH/1, without significant difference in transmission efficiency ( P =1.00). Both of the guinea pigs infected by airborne transmission of rSH/1 seroconverted; however, the one guinea pig infected by transmission of rSH/1:AN/1-NA died of anesthesia complications on day 4 post-inoculation, and thus seroconversion could not be assessed ( Table 4 ). Nevertheless, our data suggest that, although airborne transmission of H7N9 viruses in guinea pigs is inefficient overall, the acquisition of oseltamivir resistance does not further impair transmissibility. In conclusion, we have shown that the Shanghai/1-NA gene confers high-level oseltamivir resistance in vitro , but the gain of oseltamivir resistance does not attenuate virulence in mice, transmission among guinea pigs or replicative ability in either species. Severe clinical outcomes have been observed in H7N9-infected patients with delayed or ineffective viral clearance; in some cases, identification of the R292K NA inhibitor resistance mutation has been associated with persistent viral replication despite oseltamivir treatment [12] . We thus investigated the susceptibility of two representative H7N9 NAs to inhibition by three clinically available NA inhibitors, as well as the effect of oseltamivir resistance on the in vitro and in vivo replicative capacity and pathogenicity of H7N9 viruses. The arginine at position 292 (in N2 numbering, corresponding to N9 R294) is one of seven residues highly conserved among all known viral and bacterial sialidases [9] . It is critical for interaction with sialic acid [9] and with the sialic acid analogues oseltamivir, peramivir and zanamivir [18] at the enzyme’s active site. Previous studies with the N2 NA have indicated that the NA-R292K mutation not only enhances resistance to the inhibitory action of oseltamivir (and, to a lesser extent, that of peramivir and zanamivir) but also significantly impairs NA activity and virus replicative ability in vitro and in vivo [18] , [19] , [22] , [23] . Among the H7N9 NAs assessed to date, those encoding the NA-R292K substitution, like Shanghai/1, have demonstrated high-level oseltamivir resistance, mid-level peramivir resistance and low-level zanamivir resistance [24] , [25] , [26] . However, in contrast to H3N2 viruses, oseltamivir resistance appears not to compromise H7N9 replication in human respiratory tract cells or in mouse lungs [25] , [27] , [28] . Recently, the oseltamivir-sensitive H7N9 clinical isolate Anhui/1 has been shown to transmit, albeit inefficiently, among ferrets [25] , [27] , [28] , [29] , [30] , as does the contemporaneous H7N9 isolate Shanghai/1 (refs 27 , 28 ). Virus stocks grown from the Shanghai/1 clinical isolate have been found to contain a mixed population of oseltamivir-sensitive (NA-R292) and -resistant (NA-R292K) virus quasi-species, and recent studies have revealed that, in Shanghai/1, a predominantly oseltamivir-sensitive virus population can mask the presence of NA-R292K in a minority variant [25] , [26] . Thus, the similar virulence and transmission phenotypes shown by Shanghai/1 and Anhui/1 may reflect that the Shanghai/1 clinical isolate comprises a relatively small proportion of oseltamivir-resistant quasi-species. To our knowledge, it has yet to be demonstrated that the transmission of Shanghai/1 in ferrets can be specifically attributed to oseltamivir-resistant quasi-species. Importantly, we show here that a purely oseltamivir-resistant virus clone of Shanghai/1 is as virulent in mice and as transmissible in guinea pigs as one encoding the oseltamivir-sensitive Anhui/1-NA. The majority of published studies on H7N9 isolates to date have used Anhui/1 as a representative virus [25] , [27] , [28] , [29] , [30] . In our experiments, we compared the replicative, virulence and transmission phenotypes of the oseltamivir-sensitive Anhui/1-NA to the oseltamivir-resistant Shanghai/1-NA by expressing both NA genes in identical viral backbones. It should be noted that the Shanghai/1 and Anhui/1 NAs differ by two amino acids, the resistance-conferring catalytic residue R292K, as well as the N-terminal residue G39S (N9, G40S [11] ) in the membrane-proximal NA stalk. Certain NA stalk substitutions and deletions are known to affect NA sialidase activity; though most that have been studied are found in the membrane-distal stalk region [31] , [32] , [33] , our data cannot exclude the possibility that the G39S substitution exerts some effect on Shanghai/1-NA activity or viral fitness. Nevertheless, in the PR/8 background, the oseltamivir-resistant Shanghai/1-NA demonstrated an ~80% decrement in enzymatic activity and affinity for the fluorogenic substrate MUNANA, similar to impairments seen in N2 NAs encoding R292K [23] . Surprisingly, though, in H7N9 viruses, oseltamivir resistance had no demonstrable effect on viral replication or pathogenicity in mice or on transmissibility among guinea pigs. These results stand in stark contrast to oseltamivir-resistant, NA-292K-encoding influenza A(H3N2) viruses, which have demonstrated marked reductions in murine virulence and ferret transmission [17] , [19] , [22] , [34] . This discrepancy is most likely due to the different genetic backgrounds in which these NA subtypes are expressed. Even among influenza viruses of the same subtype, antiviral resistance mutations can result in strikingly different replication, virulence and transmissibility phenotypes. For example, in the N1 subtype, the NA-H274Y substitution (N2 numbering) is the most commonly found oseltamivir resistance mutation, and it has been reported to compromise the in vitro and in vivo fitness of older seasonal H1N1 strains like A/Texas/36/1991 and A/New Caledonia/20/1999 (refs 35 , 36 , 37 ). However, it has also been shown to have minimal or no effect on viral fitness in the 2009 pandemic H1N1 background [21] , [38] , [39] , [40] , and even to enhance the transmissibility of A/Brisbane/59/2007-like viruses in the guinea pig model [14] . Thus, the genetic background of human H1N1 strains appears to determine whether the NA-H274Y oseltamivir resistance mutation is harmful, neutral or beneficial to virus fitness. Our data cannot conclusively predict whether the Shanghai/1-NA, encoded in the gene constellation of a different H7N9 virus such as Anhui/1 or Shanghai/2, would facilitate or hinder virulence or transmission of the resulting reassortant. However, our experiments do suggest that a fitness penalty may not always accompany the NA-R292K substitution in emergent H7N9 viruses. Fitness in influenza A viruses is a multigenic trait. Our results clearly indicate that decreased NA enzymatic activity and substrate affinity in vitro do not invariably portend decreased viral replicative ability, virulence or transmissibility in vivo . We hypothesize that mutations in the NA gene, particularly in the enzymatic active site, alter the context of viral gene expression overall, perhaps compensating for reduced sialidase activity. In pre-2009 H1N1 viruses, for example, the NA-H274Y oseltamivir resistance mutation was shown to decrease surface expression of NA [13] . When the NA content of our 7:1 PR/8:N9 reassortant virus stocks was equivalent, the PR/8:AH/1-NA reassortant had 2–4 times more receptor-binding activity than PR/8:SH/1-NA, as measured by haemagglutination activity ( Table 2 ). Relatively more PR/8 HA may be incorporated into virions when it is paired with the AH/1-NA than with the SH/1-NA. The fivefold decrease in activity and affinity of the SH/1-NA, relative to that of the AH/1-NA, could be offset by a roughly threefold decrease in surface HA activity, resulting in indistinguishable measures of viral fitness in vitro and in vivo . While our experiments cannot yet confirm this hypothesis, they do bring to light a finding of great clinical concern: a novel influenza A virus, isolated from an infected human, was able to develop high-level oseltamivir resistance without demonstrable loss of replicative ability in vitro or of virulence or transmissibility in vivo . The prudent use of NA inhibitors in H7N9 influenza disease will be critical. In our experiments, we have shown that, at clinically relevant doses, orally administered oseltamivir does not suppress replication of the oseltamivir-resistant rSH/1 virus in the mouse lung. Oseltamivir demonstrates concentration-dependent pharmacodynamics, meaning that high peak drug concentrations at the site of infection are critical to its efficacy [41] . However, serum oseltamivir levels can be adversely affected by poor absorption from the gastrointestinal tract or impaired first-pass metabolism of the oral pro-drug [42] . World Health Organization (WHO) and US Centers for Disease Control and Prevention (CDC) guidelines have suggested that double-dose oral oseltamivir therapy or, where available, parenteral NA inhibitors, may be considered for severe avian influenza disease [4] , [43] , [44] . According to current data, intravenous zanamivir appears to maintain the best efficacy against the NA-R292K mutation [24] , [25] , [26] while achieving reliably high peak plasma concentrations [45] . However, where parenteral NA inhibitors are not yet approved for use, clinicians treating suspected or confirmed H7N9 influenza virus infection may consider initiating oseltamivir treatment at double or triple doses until an alternative agent can be obtained, given the apparent ease with which the NA-R292K mutation is selected under oseltamivir therapy [11] , [12] and the safety and tolerability profile of oseltamivir [46] , [47] . A recent randomized controlled trial failed to find clinical benefit with double-dose oseltamivir in severe influenza [48] ; however, the rationale for high-dose oseltamivir in H7N9 infection is to lessen the risk of selecting for resistant variants during treatment. Clearly, however, pre-clinical and clinical trials are needed to provide definitive guidance. Given the potentially severe hazards to human health posed by oseltamivir-resistant influenza A viruses, ongoing surveillance for the NA-R292K substitution will be critical, particularly in NA inhibitor-treated persons with H7N9 influenza disease. In summary, even though we observed significant differences in the in vitro enzymatic activity of oseltamivir-sensitive and -resistant N9 NAs, we found that the oseltamivir-resistant NA affected neither H7N9 viral replication in primary human respiratory tract cells nor morbidity or mortality in mice, compared with an isogenic virus expressing a similar oseltamivir-sensitive NA. Airborne transmission of our recombinant viruses among guinea pigs was relatively inefficient, as has generally been seen in ferrets inoculated with the Anhui/1, Shanghai/1 or Shanghai/2 clinical isolates [25] , [27] , [28] , [29] , [30] , [49] . However, of note, we observed no significant difference in transmissibility between viruses encoding the oseltamivir-sensitive Anhui/1-NA or the oseltamivir-resistant Shanghai/1-NA. Thus, unlike viruses of the H3N2 subtype, acquisition of oseltamivir resistance in the emergent H7N9 strain is accompanied by no measurable fitness cost in any of the models in which our experiments were performed. Cells 293T and MDCK cells were obtained from the American Type Culture Collection (ATCC) and were maintained either in Dulbecco’s minimal essential medium (DMEM) or in minimal essential medium (MEM; Gibco) supplemented with 10% fetal calf serum (HyClone) and penicillin–streptomycin (Gibco), respectively. Recombinant viruses were grown in 10-day-old specific-pathogen-free embryonated hen’s eggs (Charles River Laboratories) at 37 °C for 2 days. Human tracheobronchial epithelial cells (hTBE; Lonza) were differentiated by seeding them on 12-mm Transwell filters (pore size, 0.4 μm; Corning) that were coated with collagen type I from human placenta (Sigma-Aldrich) in 12-well plates (Corning). Cells were incubated with a 1:1 mixture of bronchial epithelial cell growth medium (BEGM; Lonza) and DMEM. When cells became confluent, liquid from the upper compartment was removed and cells were differentiated in an air–liquid interface for 4–6 weeks. Medium in the lower compartment was renewed every 48 h [50] . Construction of plasmids All eight viral genes of the influenza A/Shanghai/1/2013(H7N9) strain (SH/1; GISAID accession numbers EPI439486–EPI439494) were in vitro -synthesized by GeneArt Gene Synthesis (Invitrogen). Since the 5′ and 3′ noncoding regions of the SH/1 viral RNA segments had not been reported, the genes were constructed with noncoding regions corresponding to the consensus sequences of closely related influenza A viruses. The NA gene of influenza A/Anhui/1/2013(H7N9) (AH/1; EPI439509) was kindly supplied by Dr Richard Webby, St Jude Children's Hospital, Memphis, TN, USA. The viral gene segments were then subcloned into the ambisense expression vector pDZ [51] . Rescue of recombinant chimeric influenza A viruses Five recombinant influenza viruses—wild-type Shanghai/1 (rSH/1), a 7:1 reassortant between Shanghai/1 and the NA gene of Anhui/1 (rSH/1:AH/1-NA); 7:1 reassortants of A/Puerto Rico/8/34(H1N1) (PR/8) encoding the NA genes of either Shanghai/1 (rPR/8:SH/1-NA) or Anuhi/1 (rPR/8:AH/1-NA) and rPR/8:SH/1-HA/NA, a 6:2 reassortant between the PR/8 internal genes and the Shanghai/1-HA and -NA genes—were rescued from plasmid DNA [52] , [53] . The eight pDZ plasmids encoding the viral gene segments (1 μg each) were co-transfected into 293T cells with Lipofectamine 2000 (Invitrogen), according to the manufacturer’s protocol. At 24 h post-transfection, the virus-containing cell supernatant was inoculated by 29-gauge syringe into the allantoic cavities of 10-day-old embryonated chicken eggs, which were incubated at 37 °C for 2 days and then slowly cooled overnight at 4 °C. Allantoic fluid was collected by aseptically opening the allantoic cavity through the air sac and aspirating the allantoic fluid by pipette. The presence of virus in allantoic fluid was evaluated by haemagglutination of chicken red blood cells, and virus stock titres were determined by plaque assay of 10-fold dilutions of allantoic fluid in PBS on MDCK cells overlaid with 0.65% agar (Oxoid Ltd.) in MEM supplemented with 0.4% BSA, penicillin–streptomycin, 0.01% DEAE dextran and 1 μg ml −1 tosylsulfonyl phenylalanyl chloromethyl ketone (TPCK)-trypsin [54] . In vitro enzyme assays Reassortants of PR/8 encoding either the Shanghai/1-NA (rPR/8:SH/1-NA) or the Anhui/1-NA (rPR/8:AH/1-NA) were used for all in vitro assays at biosafety level (BSL)-2. For both Michaelis–Menten and NA inhibitor resistance assays, reactions were performed in 33 mM 2-(N-morpholino) ethane-sulfonic acid (MES; Sigma-Aldrich) with 4 mM calcium chloride at pH 6.6 (MES buffer), with a fluorogenic NA substrate, 2′-(4-methylumbelliferyl)-α-D-N-acetylneuraminic acid (MUNANA; Sigma-Aldrich), in 96-well plates (Corning) [14] , [55] . Relative fluorescence units (RFU) produced by cleaved MUNANA were measured with the Synergy H1 Hybrid Multi-Mode Microplate Reader and Gen5 software (BioTek). Determination of Michaelis–Menten parameters for H7N9 NAs NA content of stock 7:1 reassortant viruses rPR/8:SH/1-NA and rPR/8:AH/1-NA were quantified by western blot of serial virus dilutions, using antisera raised in mice against an influenza A(H11N9) virus as a primary antibody. Band densitometry was performed with ImageJ (NIH), and viruses were normalized to equivalent NA content by dilution in MES buffer. In 96-well plates, the normalized viruses were added to 1.67-fold dilutions of MUNANA substrate (11 concentrations ranging from 6–1,000 μM) and a twelfth control well of MES buffer without MUNANA to measure background fluorescence. Plates were incubated at 37 °C in the microplate reader, and the Gen5 software recorded the RFUs produced by catalysed MUNANA substrate every 90 s for 40 min, at excitation and emission wavelengths of 360 and 448 nm, respectively. For each MUNANA concentration, the measured RFUs (minus background fluorescence) were plotted against time to calculate reaction velocity (in RFU s −1 ) by linear regression. Michaelis–Menten parameters K m and V max were determined by non-linear regression of the MUNANA concentration versus velocity plots in Prism 6 (GraphPad Software) [14] . Two independent experiments, with three replicates per experiment, were performed, and results are expressed as an average of all replicates±s.e. Determination of H7N9 resistance to NA inhibitors Serial dilutions of stock viruses rPR/8:SH/1-NA and rPR/8:AH/1-NA were incubated in a saturating concentration of MUNANA (400 μM) for 1 h at 37 °C to obtain the 50% effective virus concentration (EC 50 ), at which half the substrate was catalysed. Viruses were then diluted to the EC 50 in MES buffer for use in a fluorometric neuraminidase inhibition assay) [14] , [55] . Three NA inhibitors, in 10-fold dilutions, were evaluated: oseltamivir carboxylate (Toronto Research Chemicals, North York, ON; 1 mM–1 pM), peramivir (MedChemexpress, Princeton, NJ; 1 mM–1 pM), or zanamivir (GlaxoSmithKline, Philadelphia, PA; 0.1 mM–0.1 pM). In 96-well plates, normalized viruses were added to 10 drug dilutions plus 2 no-drug control wells to measure uninhibited NA activity. For each drug, the plate also contained a row of no-virus control wells, including the 10 drug dilutions mixed only with MES buffer, to measure background fluorescence. Plates were incubated at room temperature for 45 min, and then MUNANA (400 μM) was added to all wells, followed by a 1-h incubation at 37 °C. Substrate conversion was stopped by the addition of 140 mM sodium hydroxide in 83% ethanol, and RFUs of catalysed MUNANA substrate were measured at excitation and emission wavelengths of 360 and 448 nm on a microplate reader. After subtracting the background fluorescence (as measured in the no-virus control wells), the NA activity at each drug concentration was expressed as a percentage of uninhibited NA activity by dividing the RFUs produced at each of the 10 drug concentrations by the average of the RFUs produced in the two no-drug control wells. The IC 50 of each drug for the SH/1 and AH/1 NAs was determined by plotting the percent of uninhibited NA activity as a function of the log 10 of the drug concentration, and the data were fit to a dose–response curve by non-linear regression in Prism 6. A minimum of six replicates per virus/drug pair were performed, and results are expressed as an average of all replicates with a 95% confidence interval (95% CI). Growth kinetics of recombinant viruses in hTBE cells Differentiated hTBE cells were infected at an MOI of 0.01 in PBS with 0.3% BSA in an air–liquid interface. Cells were subsequently cultured with BEGM in the lower compartment and incubated at either 33 or 37 °C. Viral supernatants were collected by adding 100 μl of PBS with 0.3% BSA to each well (surface area: 100 mm 2 ). Cells were incubated for 30 min, viral supernatants were collected and viral titres determined by plaque assay on MDCK cells. Animals All research studies involving the use of animals were reviewed and approved by the Institutional Animal Care and Use Committees (IACUC) of the Icahn School of Medicine at Mount Sinai and Rutgers, the State University of New Jersey. This study was carried out in strict accordance with the recommendations in the Guide for the Care and Use of Laboratory Animals of the National Research Council (8th Edition). Female BALB/c mice (6–8-week-old) were purchased from Jackson Laboratories (Bar Harbor, ME). All viral infections of mice were performed in accordance with CDC and USDA guidelines in the Animal Biosafety Level (ABSL)-3+ facility at the Icahn School of Medicine at Mount Sinai. Procedures were performed in accordance with Animal Welfare Act guidelines and approved by the Mount Sinai Institutional Animal Care and Use and Institutional Biosafety Committees. Briefly, five groups of mice ( n =5 per group) were anesthetized by intraperitoneal injection of a mixture of ketamine (100 mg kg −1 ) and xylazine (5 mg kg −1 ) and infected intranasally with one of four virus doses (10 1 , 10 2 , 10 3 or 10 4 PFU) in 50 μl of PBS with 0.3% BSA or mock-infected with 50 μl of PBS with 0.3% BSA. The mice were monitored daily for clinical signs of illness and for weight loss. Upon reaching 75% of initial body weight, animals were humanely euthanized by a lethal dose of ketamine and xylazine [56] . Kaplan–Meier survival curves were plotted in Prism 6 and compared by the log-rank test. The median mouse lethal dose (mLD 50 ) was calculated according to the method of Reed and Muench [57] , with 95% CI determined by the method of Thakur and Fezio [58] . Viral lung titres were determined by standard plaque assay on MDCK cells. Six-week-old female Hartley strain guinea pigs, weighing 400–450 g, were obtained from Charles River Laboratories (Montréal, QC). All viral infections of guinea pigs were performed in accordance with CDC and USDA guidelines in the ABSL-3 facility at the Regional Biocontainment Laboratory at Rutgers, the State University of New Jersey. Procedures were performed in accordance with Animal Welfare Act guidelines and approved by the Rutgers Institutional Animal Care and Use and Institutional Biosafety Committees. Guinea pigs were anesthetized by intramuscular injection of a mixture of ketamine (30 mg kg −1 ) and xylazine (5 mg kg −1 ) prior to phlebotomy, virus inoculation, nasal lavage and humane euthanasia by CO2 inhalation followed by bilateral thoracotomy [56] . Virus susceptibility to NA inhibitors in vivo Female BALB/c mice (6–8-week-old) were infected intranasally with 100 PFU of either rSH/1 or rSH/1:AH/1-NA in a total volume of 50 μl. Starting 1 h post infection, groups of five mice were administered one of four preparations: (1) intranasal zanamivir (GlaxoSmithKline), 25 mg kg −1 in 50 μl of PBS, twice daily for 5 days; (2) oral oseltamivir phosphate (Roche), 50 mg kg −1 in 400 μl of distilled water, twice daily for 5 days; (3) intranasal PBS, 50 μl twice daily for 5 days; or (4) distilled water orally, 400 μl twice daily for 5 days. Mice were euthanized on day 5 post infection, and virus titres in lung tissues were determined by plaque assay on MDCK cells. Airborne respiratory transmission experiments Guinea pig transmission experiments were performed with rSH/1 and rSH/1:AH/1-NA, with ABSL-3 containment, in the Regional Biocontainment Laboratory at Rutgers, the State University of New Jersey. During the experiment, ambient temperatures in the facility ranged from 67–72°F (19–22 °C), with 42–48% relative humidity. Each virus was assessed in four pairs of guinea pigs, with one virus-inoculated and one virus-exposed animal per pair. On day 0, an inoculum of 10 4 PFU of either rSH/1 or rSH/1:AH/1-NA in 300 μl was administered intranasally to four animals per group, and infected guinea pigs were then sequestered from naive animals to prevent cross-contamination. At day 1 post-inoculation, each guinea pig was individually housed in a modified 31 × 31 × 19 cm polycarbonate cage (#4, Thoren Caging Systems, Hazleton, PA), from one side of which a 20 × 10 cm opening had been cut and replaced with a panel of 1.25-cm wire mesh. The cages of one virus-inoculated and one virus-exposed guinea pig were aligned in pairs so that the wire mesh sides were directly opposed, allowing air to flow freely between cages but precluding direct contact between animals. Each inoculated-exposed guinea pig pair’s cages were placed in an isolator cabinet in a negative-pressure containment unit (Model RVB243116US6; Allentown, Inc., Allentown, NJ). On days 2, 4, 6 and 8 post infection, nasal lavages were performed by instilling a total of 1 ml of PBS into the nostrils and allowing it to drain by gravity onto a sterile Petri dish. Samples were collected into 1.5-ml tubes, centrifuged to pellet debris, and stored at −80 °C. Virus in nasal lavage specimens were titrated by plaque assay of 10-fold dilutions of thawed lavage fluid in PBS on MDCK cells, as described above [20] . Seroconversion was assessed by ELISA of pre- and post-infection serum samples from guinea pigs. In 96-well ELISA plates (4 HBX Immunoassay Plates, Immulon), 50 μl of purified 6:2 reassortant virus rPR/8:SH/1-HA/NA, at a concentration of 2 μg ml −1 in PBS, was applied to coat the well bottoms during an overnight incubation at 4 °C. Virus was removed, and plates were blocked with 5% non-fat milk in PBS for 1 h at room temperature. Plates were washed with PBS, and guinea pig sera (in fivefold dilutions between 1/30 and 1/3,750, in duplicate) were added to the plate and incubated for 1 h at room temperature. Plates were washed again with PBS and then incubated with 50 μl of a 1:2,500 dilution of alkaline phosphatase-linked anti-guinea pig secondary antibody (Abcam) for 1 h at room temperature. Plates were washed again with PBS, and 50 μl of p -nitrophenyl phosphate substrate (Invitrogen) was then added. After 30 min, the reaction was stopped with 50 μl of 0.75 N NaOH, and the plates were read at 405 nm in an ELISA plate reader (DTX 880 multimode detector; Beckman Coulter) [59] . The ELISA positivity cutoff value was determined from the pre-infection serum samples, using a 99.9% upper confidence limit, according to the method of Frey et al. [60] , and the endpoint titre was defined as the reciprocal of the highest serum dilution with OD 450 above the cutoff value. Transmission events were determined to have occurred in exposed guinea pigs with infectious virus isolated from nasal lavage specimens by plaque assay and with H7N9-specific antibodies detected in serum by ELISA. Transmission efficiencies were calculated as the number of exposed guinea pigs infected by transmission from an inoculated partner animal, divided by the total number exposed, and were compared by two-tailed Fisher’s exact test in Prism 6. How to cite this article: Hai, R. et al. Influenza A(H7N9) virus gains neuraminidase inhibitor resistance without loss of in vivo virulence or transmissibility. Nat. Commun. 4:2854 doi: 10.1038/ncomms3854 (2013).